Perturbation of sodium channel structure by an inherited Long QT Syndrome mutation The cardiac voltage-gated sodium channel (Na V 1.5) underlies impulse conduction in the heart, and its depolarization-induced inactivation is essential in control of the duration of the QT interval of the electrocardiogram. Perturbation of Na V 1.5 inactivation by drugs or inherited mutation can underlie and trigger cardiac arrhythmias. The carboxy terminus has an important role in channel inactivation, but complete structural information on its predicted structural domain is unknown. Here we measure interactions between the functionally critical distal carboxy terminus α-helix (H6) and the proximal structured EF-hand motif using transition-metal ion fluorescence resonance energy transfer. We measure distances at three loci along H6 relative to an intrinsic tryptophan, demonstrating the proximal–distal interaction in a contiguous carboxy terminus polypeptide. Using these data together with the existing Na V 1.5 carboxy terminus nuclear magnetic resonance structure, we construct a model of the predicted structured region of the carboxy terminus. An arrhythmia-associated H6 mutant that impairs inactivation decreases fluorescence resonance energy transfer, indicating destabilization of the distal–proximal intramolecular interaction. These data provide a structural correlation to the pathological phenotype of the mutant channel. Voltage-gated sodium channels open in response to membrane depolarization, providing a pathway for rapid influx of Na + that mediates action potential upstrokes in excitable tissues [1] , [2] . Within milliseconds, channels normally enter a non-conducting inactive state due primarily to occlusion of the inner mouth of the pore by the intracellular linker between domains III and IV (III–IV linker) [3] , [4] . Perturbation of Na + -channel inactivation can prolong the cellular action potential and alter cellular excitability, and has been linked to hypokalemic periodic paralysis [5] , [6] , [7] , inherited epilepsy [8] , [9] and cardiac arrhythmia [10] , [11] , [12] . In the heart, mutations in the gene coding for Na V 1.5 ( SCN5A ) have been linked to variant 3 of the congenital Long QT Syndrome (LQT3) [12] . The primary phenotype of these mutations, when examined in heterologous expression systems, is incomplete or unstable inactivation of Na + channels in response to prolonged membrane depolarization that results in channel activity that has been referred to as late or sustained Na + -channel current ( I SUS ). The first LQT3 mutation identified and characterized functionally is located within the III–IV linker, the inactivation gate [13] ( Fig. 1 ). Subsequently, mutations associated with LQT3 that disrupt inactivation have been identified and characterized throughout the channel with a large number clustered in the carboxy terminus (C-T) domain, implicating a critical role for this region in control of inactivation gating [14] , [15] , [16] , [17] , [18] , [19] . 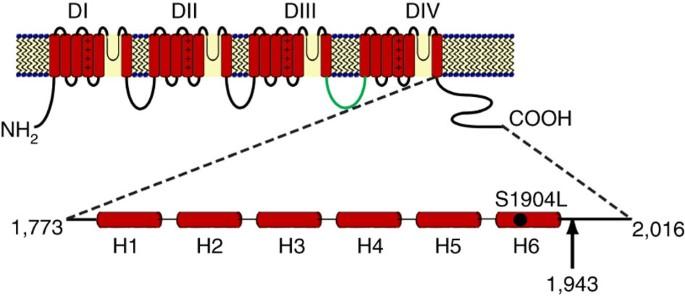Figure 1: Schematic of voltage-gated sodium channel. The four domains are designated DI, DII, DIII and DIV. The III–IV linker is shown in green. The amino and carboxy termini are designated by NH2and COOH, respectively. The C-T is expanded by six α helices (H1–H6). The approximate location of the 1,943 stop used in the constructs in this study is indicated on the expanded C-T, as well as the approximate location of the S1904L mutation. Figure 1: Schematic of voltage-gated sodium channel. The four domains are designated DI, DII, DIII and DIV. The III–IV linker is shown in green. The amino and carboxy termini are designated by NH 2 and COOH, respectively. The C-T is expanded by six α helices (H1–H6). The approximate location of the 1,943 stop used in the constructs in this study is indicated on the expanded C-T, as well as the approximate location of the S1904L mutation. Full size image An initial homology model predicted, and circular dichroism results supported, the presence of six putative helices in the amino (N)-terminal half of the C-T [20] ( Fig. 1 ). These predictions have been confirmed further by nuclear magnetic resonance (NMR) spectroscopy; the first four helices form an EF hand-like motif [21] , [22] . Biochemical and functional experiments have demonstrated interactions between the III–IV linker and the C-T that modulate inactivation and are critically dependent on the presence of the predicted sixth helix (H6) of the C-T [23] , [24] . The H6 domain also contains the calmodulin (CaM)-binding IQ motif and has been shown to have an important role in the Ca 2+ sensitivity of the channel [25] , [26] , [27] ; however, functional characterization of an LQT3 mutation located on H6 (S1904L) shows altered inactivation with no change in Ca 2+ relative to wild-type (WT) channels, indicating an additional role for the helix apart from Ca 2+ binding/sensing [24] . Despite the apparent importance of H6 in channel function, recent structural studies of the Na V 1.5 C-T do not include H6. Multiple lines of evidence, including NMR-docking studies of H6 onto the solution NMR structure of the EF-hand domain [21] , [28] suggest a functionally important interaction between the EF-hand motif and H6 that has both a Ca 2+ -dependent and structural role in channel gating [23] , [24] , [25] . Until recently, the tools available to measure short distances between locations on proteins, as we predict those between residues on the EF and H6 would be, were limited. We utilize a newly described technique, transition-metal ion fluorescence resonance energy transfer (FRET), for measuring short distances in proteins to probe this interaction [29] , [30] . The previous reports using this technique utilized cysteines labelled with fluorescent molecules as their donor. Here we reduce alteration to the native protein by taking advantage of a single endogenous tryptophan as our FRET donor. In this study, we map the location of the functionally critical distal C-T helix (H6) relative to the proximal C-T and demonstrate, for the first time, interactions between H6 and the EF-hand motif in the contiguous C-T. Additionally, by measuring distances to multiple loci on H6 and combining these data with the previously determined NMR structure, we construct an experimentally derived computational model of the entire structured C-T. Furthermore, we find that the LQT3 mutation S1904L on the H6 decreases its FRET between loci on H6 and the proximal C-T. The model predicts a steric clash in the presence of the disease-linked mutation that provides a structural correlation for the functional consequence: disrupted Na + -channel inactivation. The model provides a framework within which a number of previously reported disease-associated mutations located within the C-T can be examined. These data support a mechanism in which proper channel inactivation requires the interaction between the distal (H6) and proximal (EF-hand domain) C-T, and that disruption of this interaction affects upstream events and leads to defects in channel inactivation predisposing mutation carriers to arrhythmia. Transition metal ion FRET measurements in the C-T To employ transition-metal ion FRET to measure distances within the Na V 1.5 C-T, we needed to identify and determine the corresponding Förster distance (R 0 ) for, a donor–acceptor pair sensitive to short distances. The Na V 1.5 C-T contains a single tryptophan at residue 1798. Because tryptophan has an intrinsic fluorescence, this residue has been used previously by our lab and others [31] , [32] in fluorescence studies of the C-T. We chose to use this intrinsic tryptophan as the fluorescent donor in transition-metal ion FRET to eliminate the introduction of additional non-native residues and to improve the accuracy of the distance measurements by reducing the error attributed to linkers between cysteine-conjugated fluorophores [30] . We chose to use Ni 2+ as the fluorescent acceptor and measured the Förster distance for tryptophan and Ni 2+ as donor and acceptor to be 12 Å (Methods). We next identify a stable domain of the Na V 1.5 C-T containing the putatively structured region including the H6. Using limited proteolysis, a stable region of the C-T is determined that contains the six putative helices from amino acid residues 1773 (at the end of domain IVS6) to residue 1943 ( Fig. 1 ). This region was cloned into a bacterial protein expression vector and resulted in sufficient yields of monodisperse protein suitable for use in fluorescence spectroscopy experiments. The first experiments served two primary purposes: to validate the use of the single endogenous tryptophan as a fluorescence donor in the Na V 1.5 C-T protein; and to 'calibrate' this system by probing the distance between two points on the known EF-hand structure. The histidine pairs are chosen to be on an α-helix at any residue ( i ) and an additional residue on approximately the same face of the helix ( i +4) or ( i +3). We chose two residues on the fourth helix (H4; F1855 and K1859), based on the NMR structure, estimated to be at a distance within the detectable range of our technique to measure the FRET between the native tryptophan W1798 and a metal ion coordinated by substitution of histidines at these two residues ( Fig. 2a ). 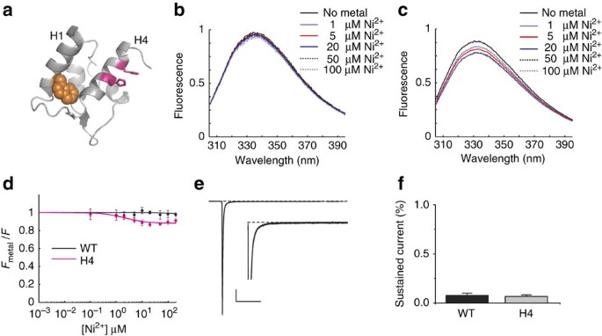Figure 2: Measurement of H4 di-histidine using transition-metal ion FRET is similar to the NMR structure and does not affect function. (a) Model of the NaV1.5 CT EF-hand domain from the solution NMR structure by Chagotet al. (2009). Introduced histidines on the fourth helix (H4) are modelled in magenta. The tryptophan on the first helix (H1) used as the fluorescence donor is modelled in orange. (b) Representative tryptophan emission dose–response spectra of NaV1.5 CT 1943 (WT) with increasing concentrations of Ni2+. (c) Representative tryptophan emission dose–response spectra of NaV1.5 CT H4 di-HIS (F1855H/K1859H). (d) Fluorescence quenching of NaV1.5 CT WT (black) and H4 di-HIS (magenta) in the presence of Ni2+. Curves are averaged-normalized fits with a modified Hill equation (seemethods). Points are averaged-normalized individual data points±s.d. (e) WT (grey) and H4-diHis (black) NaV1.5 traces shown at low gain and high gain to show absence of persistent current in both. Vertical scale bars represent 10% peak current for low-gain and 2% peak current for high-gain insets. Horizontal scale bars represent 25 ms for low-gain and 32 ms for high-gain insets (f) Introduction of H4 di-histidine mutations does not increase persistent Na current. Scale bars represent sustained current (%) to peak current at 150 ms for WT (n=7) and H4 di-HIS (n=6). Scale bars are mean±s.d. Figure 2: Measurement of H4 di-histidine using transition-metal ion FRET is similar to the NMR structure and does not affect function. ( a ) Model of the Na V 1.5 CT EF-hand domain from the solution NMR structure by Chagot et al . (2009). Introduced histidines on the fourth helix (H4) are modelled in magenta. The tryptophan on the first helix (H1) used as the fluorescence donor is modelled in orange. ( b ) Representative tryptophan emission dose–response spectra of Na V 1.5 CT 1943 (WT) with increasing concentrations of Ni 2+ . ( c ) Representative tryptophan emission dose–response spectra of Na V 1.5 CT H4 di-HIS (F1855H/K1859H). ( d ) Fluorescence quenching of Na V 1.5 CT WT (black) and H4 di-HIS (magenta) in the presence of Ni 2+ . Curves are averaged-normalized fits with a modified Hill equation (see methods ). Points are averaged-normalized individual data points±s.d. ( e ) WT (grey) and H4-diHis (black) Na V 1.5 traces shown at low gain and high gain to show absence of persistent current in both. Vertical scale bars represent 10% peak current for low-gain and 2% peak current for high-gain insets. Horizontal scale bars represent 25 ms for low-gain and 32 ms for high-gain insets ( f ) Introduction of H4 di-histidine mutations does not increase persistent Na current. Scale bars represent sustained current (%) to peak current at 150 ms for WT ( n =7) and H4 di-HIS ( n =6). Scale bars are mean±s.d. Full size image We next purified WT C-T protein (Na V 1.5 C-T 1943) and the C-T protein with the di-histidine site introduced on H4 (H4 di-HIS (Na V 1.5 C-T F1855H/K1859H)) and measured fluorescence of W1798 in the presence of increasing Ni 2+ . The fluorescence spectra ( Fig. 2b ) indicate that there is no quenching of the fluorescence of the WT protein with increasing Ni 2+ ( Fig. 2d ), whereas increasing Ni 2+ concentrations quenched H4 di-HIS Trp fluorescence emission ( Fig. 2c,d ). The quenching curve for H4 di-HIS is well fit with a modified Hill equation (Methods). The critical measurement in determining the distance is the FRET efficiency, E , which is 12±1% ( Table 1 ) for H4 di-HIS. We modelled a Ni 2+ coordinated by mutations of F1855 and K1859 to histidine within the NMR structure and measured a distance of ∼ 17 Å. The experimentally determined value between W1798 and the Ni 2+ coordinated by H4 di-HIS is 16.7±0.3 Å, in close agreement with the distance measured within the NMR structure, confirming the utility of using an intrinsic tryptophan as fluorescence donor and the accuracy of this technique relative to the NMR structure. Additionally, to assure that introduction of two histidine residues on a helix within the C-T does not significantly alter the C-T structure, the functional properties of the channel were examined. After measuring the steady-state inactivation and sustained current, we found no effect on channel inactivation properties ( Fig. 2e,f and Tables 2 and 3 ). Table 1 Summary of FRET data. Full size table Table 2 Summary of sustained current measurements. 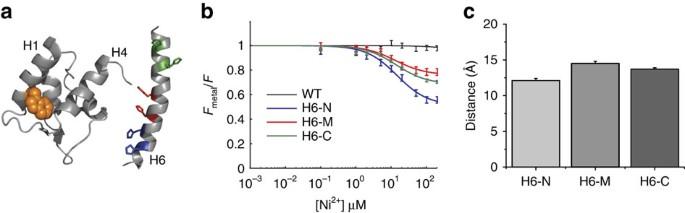Figure 3: The distance between the distal and proximal C-T measured using transition-metal ion FRET. (a) Model of the proximal (EF-hand motif) C-T is shown as inFigure 2. The H6 is shown on the right with the three di-histidine pairs: H6-N, H6-M and H6-C indicated with blue, red and green side chains, respectively. (b) Ni2+-dependent quenching of H6-N (blue), H6-M (red) and H6-C (green;Table 1). (c) Distances of H6-N, H6-C and H6-M measured using transition-metal ion FRET. Scale bars represent mean distance±s.d. of H6-N (n=4), H6-M (n=7) and H6-C (n=5). Full size table Table 3 Summary of steady-state inactivation measurements. Full size table The distal and proximal C-T are in close proximity We next sought to define the position of the H6 within the C-T structure by measuring distances between W1798 and Ni 2+ ions bound to introduced di-histidine sites along the length of H6. The first H6 di-histidine pair was introduced into the middle of H6 at positions M1906 and R1910 (H6-M; Fig. 3a ). We measured a concentration-dependent Ni 2+ -induced decrease in fluorescence ( Fig. 3b ), demonstrating close proximity between H6 and the H1 Trp. The distance calculated from the FRET efficiency ( E =24±3%, Table 1 ) is 14.5±0.3 Å ( Fig. 3c ). For further information about the orientation of H6 relative to H1, di-histidine pairs were then introduced into the C terminal (H6-C) and N terminal (H6-N) ends of the H6 helix ( Fig. 3a ). In the N terminus of H6, we tested the introduction of a histidine at V1903 to coordinate Ni 2+ binding with an endogenous histidine at position 1900 (H1900; H6-N). This protein had robust quenching ( E =49±4%; Fig. 3b ) corresponding to a distance of 12.1±0.3 Å ( Fig. 3c ) between W1798 and the Ni 2+ bound to this di-histidine. This pair would be expected to be on approximately the same face of an α-helix as H6-M. To examine the C terminal end of H6, we then mutated a glutamine at residue 1918 to pair with the native H1915. This di-histidine pair had FRET that was intermediate to that of the H6-N and H6-M ( E =31±2%), corresponding to a distance of 13.7±0.3 Å ( Fig. 3b,c ). Again, we tested the functional properties of the channel in the presence of these mutations and found no significant differences in channel function relative to the WT channels for each of the H6 histidine mutations studied ( Tables 2 and 3 ). Figure 3: The distance between the distal and proximal C-T measured using transition-metal ion FRET. ( a ) Model of the proximal (EF-hand motif) C-T is shown as in Figure 2 . The H6 is shown on the right with the three di-histidine pairs: H6-N, H6-M and H6-C indicated with blue, red and green side chains, respectively. ( b ) Ni 2+ -dependent quenching of H6-N (blue), H6-M (red) and H6-C (green; Table 1 ). ( c ) Distances of H6-N, H6-C and H6-M measured using transition-metal ion FRET. Scale bars represent mean distance±s.d. of H6-N ( n =4), H6-M ( n =7) and H6-C ( n =5). Full size image Model of proximal and distal C-T interaction The FRET distances between three distinct loci on H6 and W1798 in the EF-hand region provided us with three constraints to be used in docking calculations to generate models of the predicted structured portion of the Na V 1.5 C-T. The approach was to dock H6 on the EF-hand region using the previously reported NMR structures [21] , [22] , constrained by the FRET measurements and the constraints placed on the orientation of H6 by the rest of the C-T, followed by simulated annealing and refinement in explicit solvent to search for the lowest energy states ( Fig. 4a ). Although the docking models in the top-scoring cluster had some variability in the H5 region, the docking orientation of H6 to the rest of the channel was similar; therefore, we will use the lowest energy model to describe the model predictions. The model predicts that H6 packs against the EF hand, primarily making interactions with helices H1 and H4, burying a substantial amount of solvent-accessible surface area. In this model, the H6 overlies H1 in an anti-parallel fashion and contacts the most N-terminal region of H4. In addition, H6 also interacts with several residues in the H1–H2 and H2–H3 loops ( Fig. 4b ). It appears that the distal region of the H6, including residues R1914, H1915 and Q1918, is likely to interact with the aromatic residues F1791 and Y1795 on H1 ( Fig. 4c ), potentially stabilizing the packing interaction between the EF hand and the H6 within the C-T. 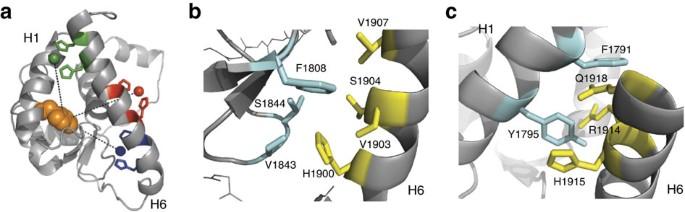Figure 4: Structural model of the NaV1.5 C-T. (a) Model of structured NaV1.5 C-T. The tryptophan (W1798) is shown as orange space-filling model. The H6 di-histidine pairs are indicated as inFigure 3with Ni2+ion coordinated by their respective di-histidine pairs shown as spheres of the same colour. The distances predicted by the model are 12.3, 15.2 and 14.1 Å for H6-N (blue), H6-M (red) and H6-C (green) di-histidines, respectively. (b) Interactions between side chains of residues on the N terminal end of H6 (H1900, V1903, S1904, V1907L denoted by yellow side chains) and side chains of residues on the H1–H2 linker (F1808, denoted by cyan side chain) and the H2–H3 linker (V1843 and S1844, also in cyan) as predicted by the model. (c) Interactions between side chains of residues at the C-T of H6 (R1914, H1915, Q1918 in yellow) and the aromatic residues on H1 (F1791 and Y1795, in cyan) also as predicted by the model. Figure 4: Structural model of the Na V 1.5 C-T. ( a ) Model of structured Na V 1.5 C-T. The tryptophan (W1798) is shown as orange space-filling model. The H6 di-histidine pairs are indicated as in Figure 3 with Ni 2+ ion coordinated by their respective di-histidine pairs shown as spheres of the same colour. The distances predicted by the model are 12.3, 15.2 and 14.1 Å for H6-N (blue), H6-M (red) and H6-C (green) di-histidines, respectively. ( b ) Interactions between side chains of residues on the N terminal end of H6 (H1900, V1903, S1904, V1907L denoted by yellow side chains) and side chains of residues on the H1–H2 linker (F1808, denoted by cyan side chain) and the H2–H3 linker (V1843 and S1844, also in cyan) as predicted by the model. ( c ) Interactions between side chains of residues at the C-T of H6 (R1914, H1915, Q1918 in yellow) and the aromatic residues on H1 (F1791 and Y1795, in cyan) also as predicted by the model. Full size image Effects of an LQT3 mutant on distal–proximal interactions With the model of the predicted structured region of the Na V 1.5 CT domain, we next turned to a previously described LQT3 mutation in H6 (S1904L) [24] and asked whether this mutation might affect the distance measurements between the tryptophan on H1 and the di-histidine pairs on H6. This mutation is of interest because it is located on the putative H6, disrupts interaction with the DIII–DIV linker and alters channel inactivation. Furthermore, our model predicts an interaction between H6 and the H1–H2 linker that would be disrupted by mutation of this residue from serine to leucine ( Fig. 5a ). The S1904L mutation was introduced into all three H6 di-histidine backgrounds and assayed for FRET. The mutation in the H6-M di-histidine background exhibited no FRET ( Fig. 5c ). This indicates that, on average, the di-histidine site in the presence of S1904L has moved beyond the range for which FRET can accurately be detected ( ∼ 20 Å), indicating a movement of >5 Å. However, the mutation in the H6-N and H6-C backgrounds resulted in 14±3 and 10±2% FRET efficiency, respectively ( Fig. 5b,d ). These measurements correspond to distances of 16.3±0.6 and 17.5±0.5 Å, respectively, suggesting an ∼ 4 Å increase in the distance between W1798 and the respective H6 di-HIS coordinated Ni 2+ ( Fig. 5f ). The S1904L in the H6-N and H6-C backgrounds was not functionally different from the S1904L mutation alone ( Fig. 5e and Tables 2 and 3 ). However, the S1904L in the H6-M background had additional disruptive effects on inactivation properties, including sustained current ( Table 2 ). Taken together, the FRET results indicate structural perturbation of the Na V 1.5 C-T proximal–distal interaction caused by the LQT3 mutation S1904L. 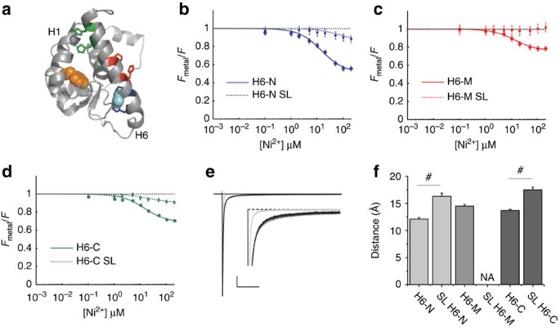Figure 5: A Long-QT Syndrome type 3 (LQT3) mutation causes a structural change. (a) Model of the NaV1.5 structured C-T as shown inFigure 4. The locus of the LQT3 mutation (S1904) is represented as a cyan space-filling side chain on H6. (b) FRET measurements for H6-N in the absence (blue solid line and circles) and presence (blue dashed line and squares) of the LQT3 mutation. (b) FRET measurements for H6-M in the absence (red solid line and circles) and presence (red dashed line and squares) of the S1904L mutation. (c) FRET measurements for H6-C in the absence (green solid line and circles) and presence (green dashed line and squares) of S1904L. The dashed black line in panels (b) through (d) represents no FRET. (e) WT (light grey), S1904L (grey) and H6-C S1904L (black) traces shown at low gain and high gain to show similarly increased late current in both S1904L and H6-C S1904L. Introduction of H6-C (Q1918H) does not affect the SL mutant phenotype. Zero shown as broken line. Vertical scale bars represent 10% peak current for low-gain and 2% peak current for high-gain insets. Horizontal scale bars represent 25 ms for low-gain and 32 ms for high-gain insets. (f) Distances measured for S1904L and H6 di-histidines in the S1904L background. Scale bars represent mean distance±s.d. of H6-N (n=4), SL H6-N (n=4), H6-M (n=7), SL H6-M (n=8), H6-C (n=5) and SL H6-C (n=4). Statistical significance (P<0.005) is denoted by #. Figure 5: A Long-QT Syndrome type 3 (LQT3) mutation causes a structural change. ( a ) Model of the Na V 1.5 structured C-T as shown in Figure 4 . The locus of the LQT3 mutation (S1904) is represented as a cyan space-filling side chain on H6. ( b ) FRET measurements for H6-N in the absence (blue solid line and circles) and presence (blue dashed line and squares) of the LQT3 mutation. ( b ) FRET measurements for H6-M in the absence (red solid line and circles) and presence (red dashed line and squares) of the S1904L mutation. ( c ) FRET measurements for H6-C in the absence (green solid line and circles) and presence (green dashed line and squares) of S1904L. The dashed black line in panels ( b ) through ( d ) represents no FRET. ( e ) WT (light grey), S1904L (grey) and H6-C S1904L (black) traces shown at low gain and high gain to show similarly increased late current in both S1904L and H6-C S1904L. Introduction of H6-C (Q1918H) does not affect the SL mutant phenotype. Zero shown as broken line. Vertical scale bars represent 10% peak current for low-gain and 2% peak current for high-gain insets. Horizontal scale bars represent 25 ms for low-gain and 32 ms for high-gain insets. ( f ) Distances measured for S1904L and H6 di-histidines in the S1904L background. Scale bars represent mean distance±s.d. of H6-N ( n =4), SL H6-N ( n =4), H6-M ( n =7), SL H6-M ( n =8), H6-C ( n =5) and SL H6-C ( n =4). Statistical significance ( P <0.005) is denoted by #. Full size image Evidence from previous studies suggest that the III–IV linker interacts with the C-T and that this interaction requires the presence of the most distal predicted C-T helix, H6 [23] , [24] . Additionally, mutation or deletion of H6 causes a disruption of the C-T/III–IV linker interface and disrupts inactivation, leading to the hypothesis that inactivation is carried out by an inactivation complex, which includes the III–IV linker and the C-T, and critically requires the presence of H6. In support of this hypothesis are clinical diagnoses of LQT3 in patients who harbour mutations in the C-T, in which these mutant channels do not completely inactivate [15] , [17] , [24] . This evidence points to the importance of the C-T, and especially H6 for proper inactivation of the channel. In addition to its structural role, H6 also has a role in calcium sensing. A recent study demonstrates that H6 binds the C-lobe of apo-CaM [33] . Previous studies demonstrate that increased calcium displaces the C-lobe of CaM from H6 to interact with the III–IV linker, as well as to increase the affinity of the EF-hand region for Ca 2+ (refs 27 , 34 ). Numerous studies have implicated H6 in interactions with the proximal C-T, the III–IV linker and even the N terminus [21] , [23] , [27] , [35] . Taken together, these studies reflect the diverse and important functional role that H6 has in channel gating. However, the location of H6 in the tertiary structure within the C-T is not known. To assist in understanding the structural role of H6 in inactivation and the pathogenesis of LQT3 mutations in the C-T, we utilized transition-metal ion FRET to measure intra-C-T interactions. To extend the method, we took advantage of a native tryptophan and, using this approach, we were able to confirm interaction between the proximal (EF-hand motif) and distal (H6) C-T at multiple loci in a polypeptide containing the entire putatively structured C-T. The results place H6 within close proximity to H1–H4 and illustrate its importance in the structure of the proximal C-T. Using these data in combination with the previously determined NMR models, we were able to construct a structural model of the C-T. The model of the C-T predicts several important interactions between H6 and the EF-hand motif in the contiguous polypeptide that provide insight into the structure–function relationship of inherited mutations. The N-terminal residues on H6 facing the EF-hand motif appear to interact with residues in the H1–H2 and H2–H3 linkers, and the C terminal residues on H6 facing the EF-hand motif appear to interact with aromatic residues on H1, particularly F1791 and Y1795. One location of particular interest is the S1904 residue examined in this and other studies. The model suggests that mutation of the serine at 1904 to leucine (S1904L), as in the LQT3 mutation, would result in a steric clash that could displace H6 relative to the EF-hand motif as indicated by the FRET measurements in the presence of this mutation. These data also provide evidence that the proximity of H6 to the EF-hand motif is important for proper inactivation. In a previous study, the LQT3 S1904L mutation was shown to have an atypical phenotype for LQT3 and to disrupt interactions between the C-T and the DIII–DIV linker. The S1904L mutation disrupts both the intra-C-T interactions, as well as the interactions between the III–IV linker and the C-T [24] . As the presence of H6 is necessary for the interaction with the III–IV linker [23] , this raises the possibility that the disruption of the H6–EF interaction in turn disrupts interactions with the III–IV linker. Interestingly, the S1904L mutation may also have an additional role in Ca 2+ sensing through disruption of CaM binding to the C-T; therefore, patients harbouring this mutation may have two types of functional consequences: the late reopenings due to disruption of the proximal–distal interaction, as well as the Ca sensitivity due to the displacement of CaM. Another residue of particular interest is the tyrosine at residue 1795 in H1 (Y1795). Y1795 has proven to be a site of multiple missense mutations leading to cardiac disease [17] , [19] . Mutations have been identified at this locus resulting not only in LQT3, but also in the Brugada Syndrome, another heritable arrhythmia generally associated with loss of Na + -channel activity, or both syndromes upon insertion of an aspartate [19] . The model predicts that this residue would closely interact with residues on H6, in particular an arginine (R1914) raising the possibility of a cation– π interaction in the WT channel, which might stabilize this interaction and consequently stabilize the inactivation process. The distance measurements from the transition-metal ion FRET place H6 closely associated with the EF-hand region of the C-T in the WT protein. If the H6 is displaced by ∼ 4 Å in the presence of the S1904L mutation, and H6 is somehow integral to the C-T/III–IV interaction, as demonstrated in previous studies, then the tertiary structure would be different and this would likely reduce the affinity of the entire C-T for the III–IV linker, as demonstrated previously with isothermal titration calorimetry and far-western blotting [24] . This may prove to be a mechanism common to mutations in this region. For example, as mentioned previously, the model predicts that the Y1795 interacts closely with an arginine at residue 1914. Mutation of Y1795 to cysteine would disrupt this interaction, and the proximal–distal C-T interaction, resulting in the late current measured experimentally. Understanding the mechanism through which disease-linked LQT3 mutations manifest their deleterious effects, the pathophysiology, requires a basic understanding of how the cardiac Na + channel functions. The work presented here examines how small perturbations in amino acids in one part of the channel, the C-T, can lead to small functional and structural effects that can have profound physiological implications. Molecular biology A stable domain of the C-T consisting of residues between 1773 and 1943 (H1–H6) was determined using limited proteolysis as described below. This region coding for these residues were amplified via PCR and cloned into a protein expression vector, pSMT3, containing a SUMO and 6×His tags. Mutations were introduced using the Quikchange mutagenesis kit (Stratagene) and all sequences were confirmed via direct sequence analysis (Genewiz). Limited proteolysis All proteins were examined with a panel of proteases: trypsin, chymotrypsin, elastase and proteinase K. Proteins were digested at various enzyme:substrate ratios (1:100, 1:1,000, 1:2,000), and samples were removed and the reaction stopped with at 0, 30 and 60 min. These samples were run on SDS–PAGE gels, bands were excised, purified and underwent matrix-assisted laser desorption-ionization time-of-flight mass spectrometry and five cycles of N-terminal protein sequencing. Protein expression and purification All constructs were transformed in DE3 (BL21) Gold competent cells. Single colonies were inoculated into small volumes of Luria-Bertani (LB) media supplemented with the appropriate antibiotic (Kanamycin for pSMT3). These cultures were used to inoculate larger volumes of Terrific Broth and grown at 37 °C with shaking to optical density 600=0.6–0.8 at which point protein expression was induced with 0.5 mM IPTG (isopropyl- β - D -thiogalactopyranoside) and shaking at 18 °C for 18–24 h. Cultures were pelleted at 6,000 r.p.m. for 15 min and pellets were placed at −80 °C. The pellets were subsequently thawed on ice and resuspended in lysis buffer containing 20 mM sodium phosphate buffer, pH 7.4, 500 mM NaCl, 20 mM imidazole, complete EDTA-free protease inhibitor tablets (Roche), 0.5 U μl −1 RNase-free DNAse (Qiagen), 2 mM MgCl 2 and 0.2 mg ml −1 lysozyme, and incubated on ice for 1 h. These lysates were snap frozen and placed at −80 °C until ready to proceed. Upon removal from −80 °C, lysates were thawed at 37 °C and sonicated briefly on ice. Lysates were cleared by ultracentrifugation (45 min at 25,000 r.p.m. ), and the supernatants were filtered through 0.22-μm filters. The supernatant was loaded on HisTrap FF (GE Biosciences) columns on an AKTA FPLC. The SUMO tag was excised from eluates by incubation overnight at 4 °C with the SUMO protease Ulp1. These digests were concentrated and buffer exchanged, reloaded on the HisTrap columns and the flowthrough (containing the target protein from which the SUMO tag was excised) was pooled, concentrated and further purified using a combination of ion-exchange and size-exclusion chromatography as indicated. The final purified protein constructs were confirmed for mass using the matrix-assisted laser desorption-ionization time-of-flight mass spectrometry and >95% purity as assessed on Coomassie blue-stained gels. Samples were taken throughout the purification process and analysed on 4–20% Tris gels and Coomassie staining. Determination of fluorescence quantum yield ( Φ F ) The quantum yield is determined for each construct by comparing the ratios of absorbance and the integral of the emission spectra relative to a fluorescent standard ( L -Trp in our assay) using the following equation: where Φ is the quantum yield, Int is the area under the emission peak (on a wavelength scale), A is absorbance at the excitation wavelength and n is the refractive index of the sample. The subscript 'R' denotes the respective values of the reference substance Calculation of Förster distance The R 0 value for tryptophan and Ni 2+ is calculated from the equation: where Φ is the quantum yield of the donor, η is the refractive index of the medium, κ is the orientation factor and J is the overlap integral of the donor fluorescence and acceptor absorbance. It is generally assumed that both the donor and acceptor are freely rotating and can undergo unrestricted isotropic motion and for that assumption, κ 2 =2/3. The refractive index, η , is assumed to be 1.4 for protein in solution. The overlap integral, J , is calculated from the equation: where f D is the normalized donor (W1798) emission spectrum determined from the equation: and ɛ A is the molar extinction coefficient of the acceptor (Ni 2+ ). The averaged and normalized emission spectra from WT (Na V 1.5 CT 1943) peptide were used to determine R 0 . The molar extinction coefficient was determined from the absorbance of Ni 2+ bound to di-histidine containing protein at a 3:1 protein/metal ratio. Fluorescence spectroscopy The purified C-T protein was diluted to a concentration of 20 μM in 10 mM HEPES buffer, pH 7.4 and 250 mM NaCl. For transition metal-binding curves, protein was mixed with an equal volume of NiSO 4 solution at various concentrations in water and kept on ice. Steady-state fluorescence emission spectra were acquired with a Fluorolog-3 fluorometer (Horiba JobinYvon). The tryptophan (W1798) was selectively excited at 295 nm and emission spectra were collected between 285 and 400 nm. The excitation and emission filter were set at 2 and 5 nm, respectively. All spectra were blank corrected, corrected for inner filter effects of metal, and normalized to the fluorescence before the addition of metals. Fluorescence data analysis Fluorescence data were collected at increasing metal concentrations and fit to a modified Hill equation to solve for K d (dissociation constant) and E (FRET efficiency): where F metal / F is the normalized fluorescence. Distance between the fluorescent Trp and the introduced metal ion is calculated using the Förster equation where R is the distance between Trp and the metal ion, and R 0 is the Förster distance, the distance at which the donor-acceptor energy transfer is 50% between tryptophan and Ni 2+ . Fluorescence data were analysed using Origin (OriginLab) and programs written in MatLab (Mathworks). Curves are averaged fits and points are the mean±s.d. Electrophysiology Mutations to pcDNA3.1 Na V 1.5 were introduced using QuikChange site-directed mutagenesis kit (Stratagene). Full-length WT or mutant Na V 1.5 was transfected into HEK293 cells using lipofectamine. Electrophysiological recordings were carried out in a whole-cell patch clamp configuration using physiological solutions. The internal solution contained 50 mM aspartic acid, 60 mM CsCl, 5 mM Na 2 -ATP, 11 mM EGTA, 10 mM HEPES, 1 mM CaCl 2 and 1 mM MgCl 2 , with pH 7.4 adjusted with CsOH. The external solution contained 130 mM NaCl, 2 mM CaCl 2 , 5 mM CsCl, 1.2 mM MgCl 2 , 10 mM HEPES and 5 mM glucose, with pH 7.4 adjusted with CsOH. Data was collected using Axopatch 200B amplifiers (Axon Instruments) and recorded with PClamp8 or 10 (Axon Instruments). Capacity current and series resistance compensation were carried out using analogue techniques according to the amplifier manufacturer (Axon Instruments). All measurements were obtained at room temperature (22 °C). Late or sustained sodium current was measured as tetrodotoxin (50 μM)-sensitive current 200 ms after depolarization to −10 mV. Statistical significance was determined using unpaired Student's t -test, P <0.05 was considered statistically significant. Computational model All docking calculations were performed with a local version of HADDOCK2.1 (ref. 36 ) or its web server implementation ( http://haddock.chem.uu.nl/services/HADDOCK/haddock.php ) [37] . The available structures of the C-T EF hand [21] (PDB ID: 2KBI ) and the H6 helix derived from a complex with Apo-CaM [33] (PDB ID: 2L53 ) were used as the starting coordinates. The docking calculations were guided with the distance restraints obtained from the FRET measurements to generate 1,000 rigid body-docking models. The 200 lowest energy models were selected for simulated annealing and further refinement in explicit solvent. The resultant lowest energy-docking model in the top-scoring cluster was then selected for the analysis. How to cite this article: Glaaser, I. W. et al . Perturbation of sodium channel structure by an inherited Long QT Syndrome mutation. Nat. Commun. 3:706 doi: 10.1038/ncomms1717 (2012).